Transmission from the dominant input shapes the stereotypic ratio of photoreceptor inputs onto horizontal cells Many neurons receive synapses in stereotypic proportions from converging but functionally distinct afferents. However, developmental mechanisms regulating synaptic convergence are not well understood. Here we describe a heterotypic mechanism by which one afferent controls synaptogenesis of another afferent, but not vice versa. Like other CNS circuits, zebrafish retinal H3 horizontal cells (HC) undergo an initial period of remodelling, establishing synapses with ultraviolet and blue cones while eliminating red and green cone contacts. As development progresses, the HCs selectively synapse with ultraviolet cones to generate a 5:1 ultraviolet-to-blue cone synapse ratio. Blue cone synaptogenesis increases in mutants lacking ultraviolet cones, and when transmitter release or visual stimulation of ultraviolet cones is perturbed. Connectivity is unaltered when blue cone transmission is suppressed. Moreover, there is no cell-autonomous regulation of cone synaptogenesis by neurotransmission. Thus, biased connectivity in this circuit is established by an unusual activity-dependent, unidirectional control of synaptogenesis exerted by the dominant input. The output of a neuron is shaped by many factors, including the properties and stereotypic patterning of the synaptic connections it receives from a diversity of cell types. Our understanding of the developmental mechanisms responsible for generating proper wiring patterns have largely come from circuits where distinct afferent types innervate separate parts of the dendritic arbour [1] , [2] . For example, hippocampal CA3 neurons are contacted by large mossy fibres on their apical dendrites, proximal to the cell body, whereas entorhinal cortical projections contact the distal dendrites [3] . A number of molecules targeting axons to the appropriate compartment of the postsynaptic cell have now been identified [4] , [5] , [6] . By contrast, we have a much more limited understanding of the mechanisms that generate stereotypic patterns of synaptic convergence in circuits where functionally distinct inputs intermingle on the dendritic arbour [7] . Here, we investigated the cellular interactions that control the connectivity of two functionally disparate presynaptic cell types whose connections overlap on the dendritic arbour of the postsynaptic cell. Like other parts of the nervous system, circuits in the vertebrate retina demonstrate a great deal of synaptic convergence and divergence [8] . Previous ultrastructural reconstructions [9] , [10] and recent light microscopy approaches [11] , [12] suggest that retinal neurons generally make a stereotypic number of synapses with each of their input types yet the mechanisms generating these patterns are not known. Complete circuit reconstruction is particularly tractable in the relatively small zebrafish retina, and many transgenic lines suitable for in vivo reconstruction are available. We focused on a simple but essential circuit in the outer retina, comprising cone photoreceptors and horizontal cells (HC), to gain an understanding of the cellular interactions responsible for setting up the appropriate synapse ratio of converging inputs. There are four types of cones in the zebrafish retina [13] , [14] , each with a peak sensitivity to either ultraviolet (UV), short (blue), medium (green) or long (red) wavelength light. In adult zebrafish, there are three types of cone HCs, classified according to their morphology and cone connectivity patterns [15] , [16] . H1 HCs contact red, green and blue cones whereas H2 HCs contact blue, green and ultraviolet cones. H1 and H2 HCs cannot be readily distinguished by their morphology. In contrast, H3 HCs can be recognized morphologically, and their circuitry is relatively simple because they contact only two cone types, ultraviolet and blue cones [16] , [17] . We show here that ultraviolet and blue cones form a stereotypic synaptic convergence ratio of about 5:1 with the H3 HCs. To determine whether the synaptic convergence ratio is dictated by the ratio of ultraviolet:blue cone number within the dendritic field of the H3 HC, we altered ultraviolet cone numbers prior to synaptogenesis with HCs, using mutant fish and morpholino approaches. To explore the role of synaptic activity in establishing the ultraviolet:blue cone synapse ratio, we generated transgenic animals in which ultraviolet or blue cone transmitter release is selectively perturbed. Because H3 HCs connect with cones largely after cone opsins are expressed, we also investigated the role of sensory experience in defining the cone connectivity pattern of H3 HCs. Together, our observations reveal a previously unknown in vivo cellular mechanism, by which one input type uses an activity-dependent process to control the number of synapses the other input type makes with their common postsynaptic partner. Morphological identification of H3 HCs during development HCs in zebrafish larval retina were labelled by expression of fluorescent protein under the Cx55.5 promoter [18] ( Fig. 1a–c ). As in adult zebrafish [15] , H1 and H2 (H1/2) cone HCs in larvae could not be readily distinguished from each other by their dendritic morphology alone, whereas H1/2 and H3 HCs appeared morphologically distinct ( Fig. 1a–c ). We found that shortly after HC genesis, H3 HCs showed lower densities of dendritic tips and larger dendritic field sizes than H1/2 HCs ( Fig. 1d ). These morphological differences persisted in older larvae ( Supplementary Fig. 1 ). As in adult zebrafish, we observed that larval HCs made invaginating dendritic contacts with cone photoreceptor axonal terminals, or pedicles. The dendritic tips of the HCs were apposed to presynaptic ribbon structures ( Fig. 1e ), and contained ionotropic glutamate receptors ( Fig. 1f ) as previously demonstrated [19] . We define here an HC-cone synapse as the invagination of a single dendritic tip within an individual cone pedicle. 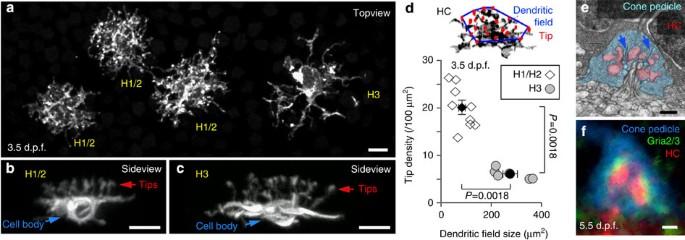Figure 1: Morphology of HCs in larval zebrafish retina. (a) Examples of HCs at 3.5 d.p.f. visualized by injecting plasmid DNA (see Methods for details) into fertilized eggs. Shown here is the maximum intensity projection of a confocal image stack of the back of an isolated eye. (b,c) Orthogonal views of two-photon reconstructions of cone HCs in live fish (3.5 d.p.f.). Dendritic tips extending from the HCs are clearly visible from these side views. Scale bars (a–c), 5 μm. (d) Tip density plotted against dendritic field size of morphologically classified H1/2 and H3 HCs at 3.5 d.p.f. The dendritic field is defined as the area encompassed by a convex polygon whose corners touch the outer most dendritic tips. Each open or grey symbol represents one cell. Black symbols and error bars represent means and s.e.m.P-values from Wilcoxon–Mann–Whitney rank sum test.n=9 for H1/2 andn=6 for H3. (e) EM image of a cone pedicle showing invaginating HC dendritic tips (red) that are apposed to characteristic presynaptic ribbons, sites of transmitter release (arrows). (f) Single plane confocal image showing Gria2/3 (also known as GluR2/3) immunoreactive puncta (green) colocalized with an HC dendritic tip (red) within a cone pedicle (blue). Scale bar (e,f), 0.5 μm. Figure 1: Morphology of HCs in larval zebrafish retina. ( a ) Examples of HCs at 3.5 d.p.f. visualized by injecting plasmid DNA (see Methods for details) into fertilized eggs. Shown here is the maximum intensity projection of a confocal image stack of the back of an isolated eye. ( b , c ) Orthogonal views of two-photon reconstructions of cone HCs in live fish (3.5 d.p.f.). Dendritic tips extending from the HCs are clearly visible from these side views. Scale bars ( a – c ), 5 μm. ( d ) Tip density plotted against dendritic field size of morphologically classified H1/2 and H3 HCs at 3.5 d.p.f. The dendritic field is defined as the area encompassed by a convex polygon whose corners touch the outer most dendritic tips. Each open or grey symbol represents one cell. Black symbols and error bars represent means and s.e.m. P -values from Wilcoxon–Mann–Whitney rank sum test. n =9 for H1/2 and n =6 for H3. ( e ) EM image of a cone pedicle showing invaginating HC dendritic tips (red) that are apposed to characteristic presynaptic ribbons, sites of transmitter release (arrows). ( f ) Single plane confocal image showing Gria2/3 (also known as GluR2/3) immunoreactive puncta (green) colocalized with an HC dendritic tip (red) within a cone pedicle (blue). Scale bar ( e , f ), 0.5 μm. Full size image H3 HCs preferentially contact ultraviolet and blue cones Adult H3 HCs only contact ultraviolet and blue cones [16] , but whether H3 HCs also demonstrate this wiring specificity during development is not known. In order to obtain the connectivity patterns of developing H3 HCs, we coinjected pCx55.5:Gal4 and pUAS:MXFP plasmids into double transgenic fish in which ultraviolet cones ( sws1:GFP (green fluorescent protein)) and blue cones ( sws2:mCherry ) express different colour fluorescent proteins (FP) under cone type-specific promoters. We obtained confocal reconstructions of H3 HCs at various larval ages, from 3.5 days post fertilization (d.p.f. ), around the onset of synaptogenesis in the outer plexiform layer (OPL) [20] , to 10 d.p.f., when visually guided behaviour is well-established [21] ( Fig. 2a ). At all ages studied, H3 HCs contacted mostly ultraviolet and blue cones ( Fig. 2b ). On average, the number of ultraviolet cones contacted by an H3 HC increased with age ( P <0.01; one-way analysis of variance (ANOVA)), whereas the number of blue cone synapses remained constant across time points ( P >0.05; one-way ANOVA) ( Fig. 2b ). 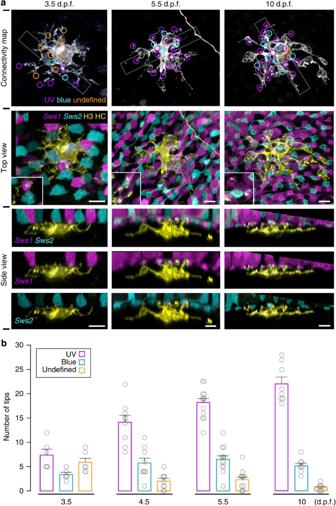Figure 2: Connectivity patterns of H3 HCs across development. (a) Examples of larval H3 HCs transiently expressing fluorescent protein in the background ofTg(sws1:GFP; sws2:mCherry). Shown are maximum intensity projections or orthogonal views through a small part of the arbour. Insets in top view panels show higher magnifications of dendritic tips invaginating into a cone pedicle. Open circles map the locations of dendritic tips that contacted ultraviolet or blue cones in the double transgenic line (magenta or blue circles respectively), as judged from 3D reconstructions of the cell and its surrounding cones. Some tips (orange circles, undefined) could not be assigned to either ultraviolet or blue cones. Scale bars, 5 μm. (b) Population data showing the mean number of ultraviolet or blue cone-associated tips and undefined tips made by H3 HCs in the background ofTg(sws1:GFP; sws2:mCherry)fish. Each open circle represents one cell.n=6 for 3.5 d.p.f.,n=9 for 4.5 d.p.f.,n=12 for 5.5 d.p.f.,n=8 for 10 d.p.f. Error bars are s.e.m. Figure 2: Connectivity patterns of H3 HCs across development. ( a ) Examples of larval H3 HCs transiently expressing fluorescent protein in the background of Tg(sws1:GFP; sws2:mCherry) . Shown are maximum intensity projections or orthogonal views through a small part of the arbour. Insets in top view panels show higher magnifications of dendritic tips invaginating into a cone pedicle. Open circles map the locations of dendritic tips that contacted ultraviolet or blue cones in the double transgenic line (magenta or blue circles respectively), as judged from 3D reconstructions of the cell and its surrounding cones. Some tips (orange circles, undefined) could not be assigned to either ultraviolet or blue cones. Scale bars, 5 μm. ( b ) Population data showing the mean number of ultraviolet or blue cone-associated tips and undefined tips made by H3 HCs in the background of Tg(sws1:GFP; sws2:mCherry) fish. Each open circle represents one cell. n =6 for 3.5 d.p.f., n =9 for 4.5 d.p.f., n =12 for 5.5 d.p.f., n =8 for 10 d.p.f. Error bars are s.e.m. Full size image We noticed that some dendritic tips were not apposed to the fluorescently labelled ultraviolet cones or blue cones, especially at 3.5 d.p.f. ( Fig. 2 , undefined tips). To determine whether fluorescent protein is not yet expressed by all ultraviolet or blue cones at early ages, we performed immunostaining with anti-ultraviolet or blue opsin antibodies. We found that at 3.5 d.p.f., 19±3% ( n =4 eyes) of ultraviolet opsin-positive cones lacked sws1:GFP expression, but by 10 d.p.f., 99±0.3% ( n =4 eyes) were visualized by GFP expression ( Supplementary Fig. 2a,b ). Almost all (>99%) blue opsin-positive cones showed sws2:mCherry expression at all ages examined ( Supplementary Fig. 2a,b ). Because of the incomplete transgene expression at early ages, the number of ultraviolet cones contacted by immature H3 HCs is likely to be greater than that quantified based on sws1:GFP labelling alone. We adjusted our measurements to account for the fraction of unlabelled ultraviolet cones, and found that the estimated number of unlabelled ultraviolet cone contacts (1.68±0.31) was still less than the average number of ‘undefined’ tips (5.83±0.87) at 3.5 d.p.f. ( Fig. 2b and Supplementary Fig. 2c ). We wondered whether some of the undefined tips were contacting red and green cones, and to test this, we performed immunostaining with the zpr-1 antibody that labels both these cone types [22] . Indeed we found that H3 HCs transiently contacted a few red and green cones before 5.5 d.p.f. ( Supplementary Fig. 3 ). Taken together, our data reveal two key characteristics of the development of cone synaptic convergence onto H3 HCs. First, elimination of red and green cone contacts contributes to the H3 HC’s mature connectivity pattern, which comprises synapses with only ultraviolet and blue cones. Second, the ultraviolet:blue cone synapse ratio increases with maturation. Selective synaptogenesis underlies ultraviolet cone dominance The synaptic bias towards ultraviolet cones may be a consequence of a greater abundance of ultraviolet cones compared with blue cones in larval zebrafish [23] . We counted the number of ultraviolet cones and blue cones present within the retina from 3.5–10 d.p.f. ( Supplementary Fig. 2a,b ), and compared these counts with the ratio of ultraviolet:blue cones that the H3 HC contacted ( Fig. 3a ). We found that the ratio of ultraviolet:blue cone synapses exceeds the relative abundance of ultraviolet and blue cones, suggesting that cone type ‘availability’ does not fully account for the biased connectivity with ultraviolet cones. 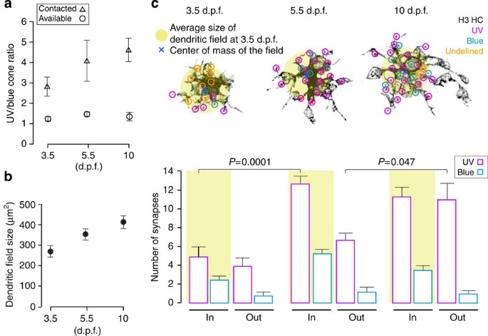Figure 3: Developmental increase in ultraviolet:blue cone synapse ratio occurs by selective addition of ultraviolet cone connections. (a) Plots across ages of the mean ratio of the ultraviolet:blue cones available (circles) as well as the adjusted mean ratio of ultraviolet:blue cones that are contacted by H3 HCs (triangles). Contacted (n=6 for 3.5 d.p.f.,n=12 for 5.5 d.p.f.,n=8 for 10 d.p.f.); available (n=4 for all ages). (b) Mean H3 HC dendritic field sizes at different ages. (c) (Upper panel) Connectivity maps of representative H3 HCs at different ages. A circle (yellow) with an area equivalent to the average 3.5 d.p.f. H3 HC dendritic field size was centred on the centre of mass of the dendritic field. (Lower panel) The mean numbers of ultraviolet and blue cone synapses within (In) or outside (Out) the yellow-filled circle were plotted for cells reconstructed at different ages. In general, synapses added outside the circle largely represent addition of synapses to the dendrites that grew after 3.5 d.p.f. In all panels, ultraviolet and blue cone synapse numbers obtained from FP expression in transgenic fish were adjusted according to the values of % transgenic expression per opsin expression fromSupplementary Fig. 2. All error bars are s.e.m.P-values from Wilcoxon–Mann–Whitney rank sum test.n=6 for 3.5 d.p.f.,n=9 for 5.5 d.p.f.,n=8 for 10 d.p.f. in (b,c). Figure 3: Developmental increase in ultraviolet:blue cone synapse ratio occurs by selective addition of ultraviolet cone connections. ( a ) Plots across ages of the mean ratio of the ultraviolet:blue cones available (circles) as well as the adjusted mean ratio of ultraviolet:blue cones that are contacted by H3 HCs (triangles). Contacted ( n =6 for 3.5 d.p.f., n =12 for 5.5 d.p.f., n =8 for 10 d.p.f. ); available ( n =4 for all ages). ( b ) Mean H3 HC dendritic field sizes at different ages. ( c ) (Upper panel) Connectivity maps of representative H3 HCs at different ages. A circle (yellow) with an area equivalent to the average 3.5 d.p.f. H3 HC dendritic field size was centred on the centre of mass of the dendritic field. (Lower panel) The mean numbers of ultraviolet and blue cone synapses within (In) or outside (Out) the yellow-filled circle were plotted for cells reconstructed at different ages. In general, synapses added outside the circle largely represent addition of synapses to the dendrites that grew after 3.5 d.p.f. In all panels, ultraviolet and blue cone synapse numbers obtained from FP expression in transgenic fish were adjusted according to the values of % transgenic expression per opsin expression from Supplementary Fig. 2 . All error bars are s.e.m. P -values from Wilcoxon–Mann–Whitney rank sum test. n =6 for 3.5 d.p.f., n =9 for 5.5 d.p.f., n =8 for 10 d.p.f. in ( b , c ). Full size image How is the bias towards ultraviolet cones established over time? The dendritic field size of H3 HCs increases with age ( P <0.02; one-way ANOVA) ( Fig. 3b ), suggesting that H3 HCs are likely to add synapses onto the distal dendrites between 3.5 and 10 d.p.f. To further assess whether the growing H3 HC arbour preferentially contacts ultraviolet cones, we compared the location of ultraviolet and blue cone contacts on the dendritic arbour of H3 HCs at different ages, as illustrated in Fig. 3c . We overlaid a circle with an area equivalent to the average dendritic field area of H3 HC dendritic arbours at 3.5 d.p.f., and compared the average number of ultraviolet and blue cone contacts within and outside this circle across ages. This circle approximates the arbour of the cell at the earliest stage examined (3.5 d.p.f. ), whereas dendrites outside the circle are likely to be added subsequently. H3 HCs added ultraviolet cone contacts within the circle up to 5.5 d.p.f., contacting nearly all of the nearby ultraviolet cones. There was no further increase in ultraviolet contacts within this circle up to 10 d.p.f. However, H3 HCs appeared to add ultraviolet cone contacts continuously to the peripheral arbour from 3.5–10 d.p.f. In contrast to ultraviolet cones, there was no addition of blue cone contacts after 5.5 d.p.f. to the peripheral arbour, suggesting that H3 HCs only form contacts with blue cones early in circuit formation. In fact, when we compared the contacts on the same cell a day apart (96 and 120 h.p.f. ), we found that ultraviolet contacts were added only to the distal dendrites ( n =3; Supplementary Fig. 4 ). Thus, preferential addition of ultraviolet cones to the peripheral arbour as the dendrites grow during later stages of development underlies the progressive increase in the ultraviolet:blue cone synapse ratio. The relatively constant number of blue cones contacted across ages may result from H3 HCs failing to attempt to form new synapses with this cone type after 3.5 d.p.f. Alternatively, H3 HCs may actively add contacts with blue cones after 3.5 d.p.f. but eliminate these contacts. To distinguish between these possibilities, we performed time lapse imaging of H3 HCs in the background of labelled ultraviolet cones ( Tg( s ws1:GFP) ) or blue cones ( Tg(sws2:GFP) ) for 24 h, beginning at 3.5 d.p.f. ( Fig. 4 ). Throughout the period of imaging, ultraviolet cone contacts were both added and eliminated ( Fig. 4a,c ), but there was a net increase in the number of ultraviolet cones contacted by the end of the recording period ( Fig. 4d ). In contrast, H3 HCs only occasionally added or eliminated blue cone contacts ( Fig. 4b,c ), resulting in almost no net change in synapses with blue cones within this time period ( Fig. 4d ). In summary, within the 24-h period of recording starting at 3.5 d.p.f., H3 HCs gained ultraviolet cone synapses, but no or relatively few blue cone contacts. Therefore, H3 HCs fail to increase their number of connections with blue cones over time because they do not actively engage blue cones in synaptogenesis after 3.5 d.p.f. 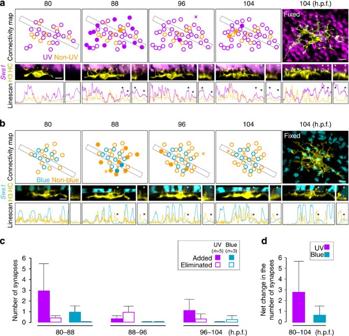Figure 4: Dynamic H3 HC processes selectively target ultraviolet cones. (a,b) Multiphoton time lapse imaging of an H3 HC in the background of (a)Tg(sws1:GFP)or (b)Tg(sws2:GFP).For each time point, an orthogonal view of the cell and labelled cones within the boxed region is provided below the connectivity map. A line scan of this region showing the relative pixel intensities of the two channels (magenta, ultraviolet cone signal or cyan, blue cone signal; yellow, HC signal) is presented below the view of the cell. Asterisks mark the location where, over time, a dendritic tip emerged and contacted ultraviolet or blue cones. Higher magnification of this location is shown on the right panels. A confocal reconstruction of the cell after fixation at the final time point (104 h.p.f.) clearly identifies the formation of new synapses. In the connectivity maps, solid circles represent synapses added in-between time points; open circles are stable contacts and X indicates eliminated contacts. Scale bars, 5 μm. (c) Population data showing the mean number of ultraviolet and blue cone synapses added and eliminated during the time course of multiphoton imaging. (d) Net change in the number of ultraviolet and blue cone synapses (n=5 for ultraviolet andn=3 for blue). Error bars are s.e.m. Figure 4: Dynamic H3 HC processes selectively target ultraviolet cones. ( a , b ) Multiphoton time lapse imaging of an H3 HC in the background of ( a ) Tg(sws1:GFP) or ( b ) Tg(sws2:GFP). For each time point, an orthogonal view of the cell and labelled cones within the boxed region is provided below the connectivity map. A line scan of this region showing the relative pixel intensities of the two channels (magenta, ultraviolet cone signal or cyan, blue cone signal; yellow, HC signal) is presented below the view of the cell. Asterisks mark the location where, over time, a dendritic tip emerged and contacted ultraviolet or blue cones. Higher magnification of this location is shown on the right panels. A confocal reconstruction of the cell after fixation at the final time point (104 h.p.f.) clearly identifies the formation of new synapses. In the connectivity maps, solid circles represent synapses added in-between time points; open circles are stable contacts and X indicates eliminated contacts. Scale bars, 5 μm. ( c ) Population data showing the mean number of ultraviolet and blue cone synapses added and eliminated during the time course of multiphoton imaging. ( d ) Net change in the number of ultraviolet and blue cone synapses ( n =5 for ultraviolet and n =3 for blue). Error bars are s.e.m. Full size image H3 HCs increase connections with excess ultraviolet cones To gain insight into the cellular interactions that regulate the balance of inputs amongst different cone types onto the H3 HC, we first asked whether increasing the density of ultraviolet cones in the retina affects their connectivity with H3 HCs. We therefore analysed H3 HC connectivity in animals in which a morpholino directed against thyroid hormone receptor β2 ( thrb morphant) causes a doubling in ultraviolet cone density without changing blue cone density [24] ( Fig. 5a–d ). 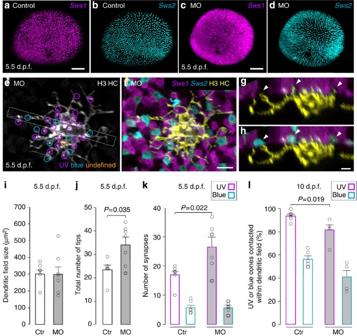Figure 5: Increasing ultraviolet cone availability leads to more ultraviolet cone synapses without affecting blue cone synapse number. (a–d) Maximum intensity projections of confocal image stacks of whole mount eyes in the background ofTg(sws1:GFP; sws2:mCherry). Ultraviolet and blue cone distributions are shown for standard morpholino-injected animals (a,b; control) and inthrbmorphants (MO). Scale bars, 50 μm. (e–h) Example of an H3 HC visualized inthrbMO, and its connectivity map. Arrowheads in the oblique view of the cell (g,h) indicate dendritic tips invaginating blue cones. Scale bars, 5 μm. (i–l) Population data comparing mean measurements in control (ctr) andthrbMO. See Methods for details of analysis. Each open circle represents one H3 HC. Error bars are s.e.m.P-values from Wilcoxon–Mann–Whitney rank sum test. Figure 5e–h shows an example of an H3 HC and its connectivity in the thrb morphant retina at 5.5 d.p.f. Compared with controls, H3 HCs in the morphant increased their total number of dendritic tips, without changing their dendritic field size ( Fig. 5i,j ). The increase in total tip number was driven by an increase in synapses with ultraviolet cones ( Fig. 5k ). By 10 d.p.f, morphant H3 HCs contacted the majority of the ultraviolet cones within their dendritic fields, as in wild-type animals ( Fig. 5l ). Thus, the number of ultraviolet cones an H3 HC contacts is dependent on the number of available ultraviolet cones within the cell’s vicinity. Despite significantly increasing their contact with ultraviolet cones, morphant H3 HCs contacted the same number of blue cones as morpholino controls ( Fig. 5k ). Therefore, during normal development, H3 HCs do not contact blue cones simply because there are insufficient ultraviolet cones available for attaining a desired total synapse number. Figure 5: Increasing ultraviolet cone availability leads to more ultraviolet cone synapses without affecting blue cone synapse number. ( a – d ) Maximum intensity projections of confocal image stacks of whole mount eyes in the background of Tg(sws1:GFP; sws2:mCherry) . Ultraviolet and blue cone distributions are shown for standard morpholino-injected animals ( a , b ; control) and in thrb morphants (MO). Scale bars, 50 μm. ( e – h ) Example of an H3 HC visualized in thrb MO, and its connectivity map. Arrowheads in the oblique view of the cell ( g , h ) indicate dendritic tips invaginating blue cones. Scale bars, 5 μm. ( i – l ) Population data comparing mean measurements in control (ctr) and thrb MO. See Methods for details of analysis. Each open circle represents one H3 HC. Error bars are s.e.m. P -values from Wilcoxon–Mann–Whitney rank sum test. Full size image Ultraviolet cone depletion increases H3 connectivity with blue cones We next asked whether decreasing ultraviolet cone density during development would affect the H3 HC’s connectivity pattern. We crossed the lots-of-rods ( lor ) mutant, in which the total number of ultraviolet cones in the retina is reduced without changing the total number of blue cones [25] , into the background of the double transgenic, Tg(sws1:GFP; sws2:mCherry) ( Fig. 6a–d ). In the lor mutant, the few remaining ultraviolet cones appear in random patches across the retina ( Fig. 6c ). An example of an H3 HC and its connectivity pattern in the mutant at 5.5 d.p.f. is provided in Fig. 6e–h . There were no significant differences in H3 HC dendritic field size between the mutant and wild-type animals ( Fig. 6i ). However, H3 HCs increased contact with blue cones ( Fig. 6k ), resulting in only a small decrease in their total contact number compared with controls ( Fig. 6j,k ). H3 HCs thus contacted a significantly higher fraction of blue cones within their dendritic fields in the lor mutant ( Fig. 6l ). 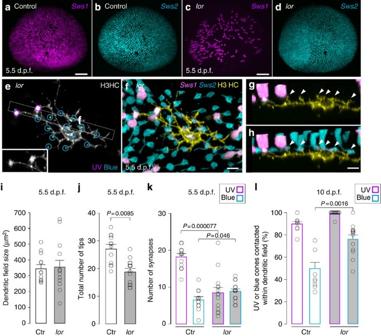Figure 6: H3 HCs increase synaptogenesis with blue cones in the absence of ultraviolet cones. (a–d) Maximum intensity projections of confocal image stacks of whole mount eyes in the background ofTg(sws1:GFP; sws2:mCherry). Ultraviolet and blue cone distributions are shown for wild-type animals (a,b; control) and in thelormutant(lor). Scale bars: 50 μm. (e–h) Example of an H3 HC visualized inlor, and its connectivity map. Inset in (e) shows a higher magnification view of enlarged dendritic tips within ultraviolet cones. Arrowheads in the orthogonal view of the cell (g,h) indicate dendritic tips invaginating blue cones. Scale bars, 5 μm. Note that inFig. 7, some ultraviolet cones inlorreceive more than one dendritic invagination from the same HC. We counted these tips as a separate ‘synapse’. (i–l) Summary of mean measurements in control (ctr) andlor. See Methods for details of analysis. Each open circle represents one H3 HC. Error bars are s.e.m.P-values from Wilcoxon–Mann–Whitney rank sum test. Figure 6: H3 HCs increase synaptogenesis with blue cones in the absence of ultraviolet cones. ( a – d ) Maximum intensity projections of confocal image stacks of whole mount eyes in the background of Tg(sws1:GFP; sws2:mCherry) . Ultraviolet and blue cone distributions are shown for wild-type animals ( a , b ; control) and in the lor mutant (lor ). Scale bars: 50 μm. ( e – h ) Example of an H3 HC visualized in lor , and its connectivity map. Inset in ( e ) shows a higher magnification view of enlarged dendritic tips within ultraviolet cones. Arrowheads in the orthogonal view of the cell ( g , h ) indicate dendritic tips invaginating blue cones. Scale bars, 5 μm. Note that in Fig. 7 , some ultraviolet cones in lor receive more than one dendritic invagination from the same HC. We counted these tips as a separate ‘synapse’. ( i – l ) Summary of mean measurements in control (ctr) and lor . See Methods for details of analysis. Each open circle represents one H3 HC. Error bars are s.e.m. P -values from Wilcoxon–Mann–Whitney rank sum test. Full size image Like in wild-type, H3 HCs in lor contacted nearly 100% of the available ultraviolet cones, but each H3 HC in lor experienced variable densities of ultraviolet cones within their dendritic field. In some cells, the dendritic tips that invaginated ultraviolet cones were enlarged ( Fig. 6e ), whereas in other cases, H3 HCs projected two tips into the same ultraviolet cone ( Fig. 7a–c ). A plot of the number of ultraviolet cone versus blue cone synapses for individual cells in lor at 5.5 d.p.f. ( Fig. 7d ) shows that in lor , there is an inverse relationship between the number of ultraviolet cones contacted and the number of blue cones contacted. Thus, H3 HCs respond to a lack of ultraviolet cones by modifying their dendritic contact area with available ultraviolet cones and by increasing their blue cone synapse number. 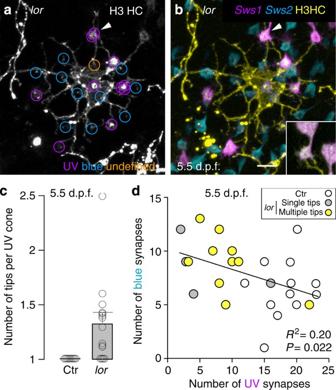Figure 7: Inverse correlation between the number of ultraviolet and blue cones synapsing with H3 HCs inlor mutants. (a,b) An example of an H3 HC labelled inTg(sws1:GFP; sws2:mCherry)crossed in thelorbackground. Connectivity map is shown in (a). Arrowhead indicates an unusual invagination into a ultraviolet cone by two dendritic tips from the same HC. Dendritic tips of larval H3 HCs normally do not show such branching or co-innervation of the same pedicle. Scale bar, 5 μm. The inset shows a high magnification view of the tip indicated by the arrowhead. (c) Quantification of the mean number of dendritic tips invaginating a single ultraviolet cone in wild-type (ctr) andlor. Open circles represent the average value for individual H3 HCs. Error bars are s.e.m. (d) The number of blue and ultraviolet cones synapsing onto a given H3 HC (each circle) at 5.5 d.p.f. are plotted here for wild-type animals (ctr) andlormutants. All control H3 HCs had a single dendritic invagination into a cone pedicle. Inlor, however, some H3 HCs project two or more dendritic tips into the cone pedicle (multiple tips).R2andP-value from Pearson correlation coefficient. Figure 7: Inverse correlation between the number of ultraviolet and blue cones synapsing with H3 HCs in l or mutants. ( a , b ) An example of an H3 HC labelled in Tg(sws1:GFP; sws2:mCherry) crossed in the lor background. Connectivity map is shown in ( a ). Arrowhead indicates an unusual invagination into a ultraviolet cone by two dendritic tips from the same HC. Dendritic tips of larval H3 HCs normally do not show such branching or co-innervation of the same pedicle. Scale bar, 5 μm. The inset shows a high magnification view of the tip indicated by the arrowhead. ( c ) Quantification of the mean number of dendritic tips invaginating a single ultraviolet cone in wild-type (ctr) and lor . Open circles represent the average value for individual H3 HCs. Error bars are s.e.m. ( d ) The number of blue and ultraviolet cones synapsing onto a given H3 HC (each circle) at 5.5 d.p.f. are plotted here for wild-type animals (ctr) and lor mutants. All control H3 HCs had a single dendritic invagination into a cone pedicle. In lor , however, some H3 HCs project two or more dendritic tips into the cone pedicle (multiple tips). R 2 and P -value from Pearson correlation coefficient. Full size image Ultraviolet cone transmission regulates connections with blue cones Our finding of a compensatory increase in blue cone contacts in the lor mutant suggests that the H3 HC’s dominant partner type, ultraviolet cones, influence connectivity with the secondary partner type, blue cones. Is this regulation mediated by transmission from cones? To test this possibility, we generated transgenic fish in which tetanus toxin fused to cyan fluorescent protein (TeNT-CFP) is expressed in ultraviolet, blue or both cone types, without changing their densities ( Supplementary Fig. 5a ). TeNT perturbs exocytosis [26] and thus reduces synaptic transmission. 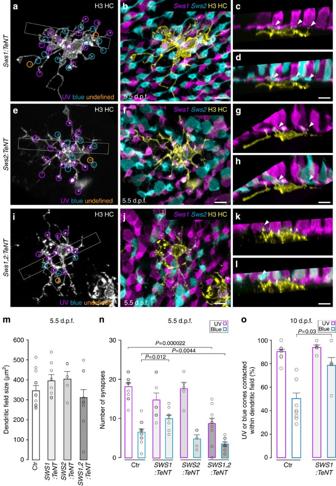Figure 8: Ultraviolet cone transmission regulates blue cone synapse number. (a–l) Examples of H3 HCs and their connectivity maps in the background ofTg(sws1:TeNT; sws2:mCherry)(a–d),Tg(sws1:GFP; sws2:TeNT)(e–h), orTg(sws1:TeNT; sws2:TeNT; sws2:mCherry)(i–l). Side views of rectangular regions outlined in (a,e,i) are shown in (c,d,g,h,k,l). Arrowheads indicate blue cone synapses. Scale bars, 5 μm. (m–o) Comparison of mean measurements across conditions. See Methods for details of analysis. Control (wildtype) animals (ctr). Each open circle represents one H3 HC. Error bars are s.e.m.P-values from Wilcoxon–Mann–Whitney rank sum test. Figure 8a–l shows an example of an H3 HC and its connectivity pattern at 5.5 d.p.f. from each of the TeNT transgenic lines. Reduction in transmission from ultraviolet, blue or both cone types did not affect the dendritic field size of H3 HCs relative to controls ( Fig. 8m ). Figure 8: Ultraviolet cone transmission regulates blue cone synapse number. ( a – l ) Examples of H3 HCs and their connectivity maps in the background of Tg(sws1:TeNT; sws2:mCherry) ( a – d ), Tg(sws1:GFP; sws2:TeNT) ( e – h ), or Tg(sws1:TeNT; sws2:TeNT; sws2:mCherry) ( i – l ). Side views of rectangular regions outlined in ( a , e , i ) are shown in ( c , d , g , h , k , l ). Arrowheads indicate blue cone synapses. Scale bars, 5 μm. ( m – o ) Comparison of mean measurements across conditions. See Methods for details of analysis. Control (wildtype) animals (ctr). Each open circle represents one H3 HC. Error bars are s.e.m. P -values from Wilcoxon–Mann–Whitney rank sum test. Full size image However, the number of blue cones contacted by an H3 HC significantly increased when only ultraviolet cone transmission was perturbed ( Fig. 8n ). This resulted in a reduction in the ultraviolet:blue synapse ratio ( Supplementary Fig. 6 ) and a larger percentage of blue cones within the field being contacted ( Fig. 8o ), similar to lor mutants ( Fig. 6l ). In contrast to lor mutants, H3 HCs maintained the same number of ultraviolet cone connections in sws1:TeNT retina as in control retina. Suppression of blue cone transmission alone did not alter the number of ultraviolet cone or blue cone contacts ( Fig. 8n ). Together, these manipulations of neurotransmission demonstrate that ultraviolet cone transmission regulates H3 HC connectivity with blue cones, but not with the ultraviolet cones themselves, and that blue cone transmission is not required for normal circuit formation. Moreover, in the absence of drive from either of the preferred cone inputs, H3 HCs do not reach out to zpr-1-immunopositive red or green cones ( n =8; sws1:TeNT , n =5; sws2:TeNT ), suggesting that partner choice is not dependent on neurotransmission from photoreceptors. However, when transmission from both ultraviolet and blue cones is suppressed, H3 HCs do show reduced contact with both cone types ( Fig. 8n ). To ascertain whether the effects of ultraviolet cone transmission are light dependent, we designed a morpholino against ultraviolet opsin ( Opn1sw1 ), rendering ultraviolet cones insensitive to ultraviolet light but allowing them to release neurotransmitter. Injection of Opn1sw1 morpholino into single-cell fertilized eggs abolished all Opn1sws1 immunoreactivity but did not affect ultraviolet cone density ( Supplementary Fig. 5b ). As in Tg(sws1:TeNT) fish, H3 HCs in the Opn1sw1 morphant demonstrated an increase in blue cone contact number without changing ultraviolet cone connectivity ( Fig. 9 ), indicating that light-dependent transmission from ultraviolet cones normally modulates synapse number with blue cones. 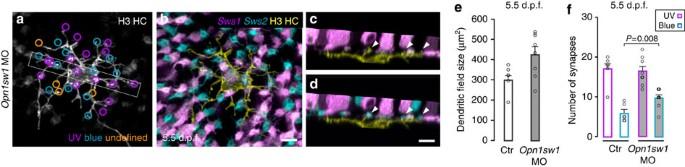Figure 9: Ultraviolet light-driven transmission regulates H3 HC connectivity with blue cones. (a–d) An H3 HC and its connectivity map in the background of aTg(sws1:GFP; sws2:mCherry)fish that was injected with a morpholino against ultraviolet opsin (Opn1sw1MO). Arrow heads indicate blue cone synapses. Scale bars, 5 μm. Comparison of measurements between standard morpholino (ctr) andOpn1sw1morpholino-injected animals. Each open circle represents one H3 HC. (e,f) Comparison of mean measurements across conditions. Control animals (ctr). See Methods for details of analysis. Each open circle represents one H3 HC. Error bars are s.e.m.P-values from Wilcoxon–Mann–Whitney rank sum test. Figure 9: Ultraviolet light-driven transmission regulates H3 HC connectivity with blue cones. ( a – d ) An H3 HC and its connectivity map in the background of a Tg(sws1:GFP; sws2:mCherry) fish that was injected with a morpholino against ultraviolet opsin ( Opn1sw1 MO). Arrow heads indicate blue cone synapses. Scale bars, 5 μm. Comparison of measurements between standard morpholino (ctr) and Opn1sw1 morpholino-injected animals. Each open circle represents one H3 HC. ( e , f ) Comparison of mean measurements across conditions. Control animals (ctr). See Methods for details of analysis. Each open circle represents one H3 HC. Error bars are s.e.m. P -values from Wilcoxon–Mann–Whitney rank sum test. Full size image It has long been appreciated that heterosynaptic modifications occur in CNS circuits in which functional changes in one input affect other inputs sharing the same postsynaptic cell [27] , [28] , [29] . Most of these past studies have focused on functional plasticity of mature synapses. Here, we show that in a developing retinal circuit, one input type regulates synaptogenesis of the other input through an activity-dependent, sensory-driven mechanism (results summarized in Supplementary Fig. 6 ). Unlike synaptic plasticity in most circuits, the regulation of synaptogenesis is unidirectional, that is, ultraviolet cone input on H3 HCs controls HC connectivity with blue cones, but not vice versa. Our analysis suggests that the stereotypic connectivity of H3 HCs is established during development through two processes. First, early in development, H3 HCs contact inappropriate partner types (red and green cones) in addition to ultraviolet and blue cones, but such errant contacts are rapidly eliminated. In this regard, H3 HCs establish specificity through an early phase of circuit refinement, which is also found in other vertebrate retinal circuits [30] as well as in many parts of the nervous system [31] , [32] . The second phase of synaptogenesis commences at the onset of cone transmission, around 3 d.p.f. [33] , and during this stage the synapse ratio of ultraviolet:blue cones increases significantly. This bias arises from H3 HCs selectively forming synapses with ultraviolet cones while maintaining synapses with blue cones that were formed early on. Many other systems establish their mature connectivity patterns by pruning inappropriate connections and further refine by eliminating some connections with appropriate partners [28] , [31] . In contrast, H3 HCs achieve their biased connectivity towards ultraviolet cones largely by selectively increasing synaptic contact with ultraviolet cones, rather than by pruning excessive blue cone contacts. The developmental increase in contact with ultraviolet cones cannot be accounted for by addition of newly generated ultraviolet cones within the field of the HC dendritic arbour because cone genesis is complete prior to synaptogenesis with H3 HCs [20] , [34] . It is also unlikely that the relative availability of presynaptic cell types alone dictates H3 HCs’ selective synapse formation with ultraviolet cones. Although ultraviolet cones outnumber blue cones by 1.5:1 at all larval stages examined, this ratio is far below the ultraviolet:blue cone synapse ratio of 5:1. Thus, H3 HCs increase synaptogenic preference for one of their two input types in the context of a stable population of presynaptic partners. Mutant fish and morpholino approaches allowed us to investigate how the relative numbers of ultraviolet and blue cones prior to synapse formation impact the convergence ratio of the presynaptic partner types. Normally, an H3 HC connects with almost all of the ultraviolet cones within its dendritic field. However, observations based on the thrb morphants suggest that H3 HCs can increase the number of synapses they make with ultraviolet cones when more ultraviolet cones are available during development. This observation resembles previous findings in nrl knockout mice in which an excess of cones develop in the absence of rods, and the HCs increase their density of synaptic contact with cones [35] . Thus, across species, the number of available presynaptic partners can set the upper limit of the number of connections they form with the postsynaptic cell. However, in zebrafish, this does not apply to synapses with secondary inputs because H3 HCs normally contact only about half of the blue cones within their dendritic fields. We found that the availability of the dominant input type can also affect the connectivity of the secondary input type. Connectivity with blue cones increases above normal levels when ultraviolet cone numbers are decreased, as in the retinas of the lor mutants. Compensatory changes in one input type when the other type is absent have been previously observed. Notably, degeneration of parallel fibres results in the expansion of the dendritic territory occupied by climbing fibres on Purkinje cell dendrites, and vice versa [36] , [37] , [38] . Is this compensatory change aimed at reaching a fixed, total number of synapses? We do not find support for this mechanism in cone-H3 HC circuits, because the total number of synapses in the thrb morphant exceeds the control number. This suggests that in wild-type animals, the number of blue cone synapses is not regulated by a mechanism that sets the total number of synapses. Instead, blue cone synapse numbers are normally maintained at low levels, but can be increased when there are fewer favored synaptic partners available to H3 HCs. Finally, the number of blue cone contacts in the thrb morphant may remain unaltered because H3 HCs in the thrb morphant increase contact with supernumerary ultraviolet cones largely after synaptogenesis with blue cones. A well-accepted mechanism that shapes neuronal connectivity patterns is activity-dependent competition [39] , [40] , [41] . Competition results in a ‘winner take-all’ scenario, in which connections with one input type are eliminated and synaptic territory is taken over by the other input type. Generally, the input that is relatively less active loses. Here, we showed that perturbing transmission from ultraviolet cones results in an increase in connectivity with blue cones, revealing an activity-dependent process. But, unlike activity-driven competitive mechanisms, the suppressed ultraviolet cones do not lose connectivity with the postsynaptic cell. This result resembles that observed when input from parallel fibres to Purkinje cells is blocked: the number of climbing fibres contacting the Purkinje cell is increased, but synapses with parallel fibres are maintained [42] . When climbing fibre input is perturbed instead, parallel fibres increase their innervation of the proximal dendrites of the Purkinje cells [43] . Together, these observations suggest that there is bidirectional influence on connectivity by both input types. In contrast, connections on H3 HCs are influenced unidirectionally by the activity of only one input; blocking blue cone transmission does not result in an increase in ultraviolet cone connectivity. Thus, we have uncovered a previously unknown mechanism that regulates the pattern of synaptic convergence onto an individual neuron, which engages an activity-dependent process that is dictated by only one afferent type, the dominant input. Why does ultraviolet cone transmission affect blue cone connectivity and not vice versa? An obvious explanation is that ultraviolet cones provide the majority of the net photoreceptor drive onto H3 HCs. When synaptic drive is diminished, either by loss of ultraviolet cones or lack of ultraviolet cone transmission, H3 HCs may seek connections with other active cones as part of a compensatory response. Thus, loss of drive from the few blue cones would not be sufficient to trigger a compensatory response. Congruent with this hypothesis, a previous study of mixed hippocampal neuronal cultures from wild-type and mutant animals lacking the NMDA receptor subunit GluN1 demonstrated the presence of a threshold (>50% inactive), only above which changes in connectivity were detected [44] . It is not clear, however, that a set threshold exists for the H3 HC-cone circuit because we find an inverse relationship between the number of blue cones and ultraviolet cones that are contacted by an individual H3 HC ( Fig. 7d ). We propose that the most parsimonious explanation is that specific loss of transmission from ultraviolet cones triggers a mechanism to recruit blue cone connections. We also noted that when all drive to H3 HCs is suppressed, both ultraviolet and blue cone connections decline. This is reminiscent of findings in mammalian retina, where blockade of transmission from all depolarizing ON-type bipolar cells leads to an overall decrease in synaptic contact with ON-type retinal ganglion cells [45] . Thus, a compensatory increase in connectivity with presynaptic cells may only occur when there are presynaptic partners that are still able to transmit. As yet, our experiments do not directly reveal whether or not the postsynaptic cell mediates the heterotypic regulation of cone connectivity. It is known that photoreceptors are coupled by gap junctions [46] , and thus the relevant signals may be conveyed directly between cones. However, if the suppressive signal passes between cones via gap junctions, then we would not expect changes to blue cone connectivity in the sws1:TeNT retina, in which we interfered with the release of neurotransmitter without preventing the cones from responding to changes in illumination. Therefore, it is more likely that transmission from ultraviolet cones acts via a mechanism directly involving the H3 HC. Indeed, in cerebellar circuits, it has been shown that Purkinje cells mediate the interactions between climbing fibres and parallel fibres that establish their respective synaptic territories [28] . Regardless of the exact ‘postsynaptic’ mechanism, our study clearly shows that synaptic convergence of each distinct input onto a sensory neuron is not necessarily independently regulated; instead, one input type can unidirectionally regulate the connectivity of the other input. Transgenic and mutant zebrafish Zebrafish were maintained and experiments conducted in accordance with University of Washington Institutional Animal Care and Use Committee guidelines. Fish were raised in an incubator with a transparent door in a room with a normal light cycle, typically lights on from 9:00 to 23:00. We used a combination of transgenic lines to visualize ultraviolet and/or blue cones by fluorescent protein (FP) expression. Tg(sws1:GFP ) [47] labels ultraviolet cones, and Tg(sws2:GFP ) [48] labels blue cones. As an additional method to visualize blue cones, a transgenic line was engineered to express mCherry in blue cones Tg(sws2:mCherry) [49] . To block neurotransmission from cones, we generated transgenic lines in which tetanus toxin light chain (TeNT) fused to CFP is expressed in ultraviolet ( Tg(sws1:TeNT) ), or blue cones ( Tg(sws2:TeNT) ). Transgenic lines were generated by plasmid injection with or without transposase RNA into fertilized eggs at the one-cell stage, and subsequent F1 generations were screened by FP expression. For in vivo time lapse imaging of the retina, we used the roy orbison mutant background [50] in which iridophores do not form. The cone innervation pattern of H3 HCs in the roy orbison mutant resembles that of wild-type fish ( Supplementary Fig. 7 ). The lor mutant was isolated from N -ethyl- N -nitrosourea-induced mutant fish [25] . Homozygous lor mutant fish showed no obvious morphological phenotype except a decreased number of ultraviolet cones and an increased number of rod photoreceptors. Plasmid generation To visualize individual HCs, we used the pCx55.5:Gal4VP16 plasmid together with plasmids that express fluorescent protein tagged with membrane localization signal under the UAS promoter (pUAS:MXFP) [51] . MXFP represents MtdCerulean, MYFP or MtdTomato. pUAS:MtdCerulean plasmid was generated by inserting a tandem repeat Cerulean coding region tagged with membrane localization signal under the UAS promoter. pUAS:MtdTomato plasmid was generated by replacing the YFP coding region from pUAS:MYFP plasmid with tdTomato. To generate transgenic fish lines, we constructed pSws1:TeNT and pSws2:TeNT plasmids using the Gateway (Life Technologies) and Tol2 system [52] . Cone type-specific promoters were excised from sws1:GFP [47] and sws2up3.2kb:EGFP plasmids [48] , and inserted into p5E plasmids. TeNT-CFP [45] was inserted into pME plasmid. Subsequent plasmids were subjected to a Gateway reaction together with p3E-polyA and pDestTol2pA. Morpholinos Morpholino sequences are 5′-CCTCTTACCTCAGTTACAATTTATA-3′ (standard control), 5′-CGAATTGAACGGCCCACGCGTCCAT-3′ ( Opn1sw1, Acc#; AF109373.1) and 5′-TCTAGAACTTGCAATACCTTTCTTA-3′ ( thrb , Acc#; AB759513). Plasmid and morpholino injection Plasmid and/or morpholino (Gene Tools, LLC) were diluted in 1 × Danieau’s solution (58 mM NaCl, 0.7 mM KCl, 0.6 mM Ca(NO 3 ) 2 , 0.4 mM MgSO 4 , 5 mM HEPES, pH 7.6) with 0.1% phenol red to aid visualization of the injection bolus. Plasmid and/or morpholino solutions were injected into fertilized eggs at the one-cell stage. A pulled-glass micropipette loaded with injection solution was attached to a Picospritzer II (Parker) and anchored on a micromanipulator (Narishige) for small volume microinjections. Injection pressure was set to 10 psi and durations ranged from 100–300 ms. Total concentrations from 20–100 ng μl −1 for plasmids with and without 0.25 mM morpholino were injected. Injected eggs were maintained in 0.3 × Danieau’s in an incubator at 28 °C. At 12–24 h.p.f., the medium was replaced with 0.3 × Danieau’s containing 0.2 mM phenylthiourea (PTU) to prevent melanin synthesis. Embryos were maintained in this medium up to 5.5 d.p.f. For the following incubation, fish were raised without PTU and fed regularly. In vivo imaging Embryos at various stages were anaesthetized with MS-222 (25–50 mg l −1 ) in 0.3 × Danieau’s solution) and mounted in molten 0.5% low-melting-point agarose (type VII, Sigma) in 60 mm organotypic culture dishes (Falcon). After solidification of the agarose, fish were covered with 0.3 × Danieau’s solution containing 0.2 mM PTU and MS-222 (25–50 mg ml −1 ). Image stacks were acquired on a confocal microscope (FV1000, Olympus) or a custom-built two-photon microscope consisting a Ti-Sapphire tunable infrared laser (Spectra-Physics) at 850–915 nm. A 1.1 NA × 60 water immersion objective lens with a refractive index correction collar was used (Olympus). Images were typically acquired with an XY resolution of 0.077 μm per pixel and 0.3 μm-thick Z slices. For time lapse imaging, zebrafish embryos were released from agarose after each image acquisition period and returned to fish water without MS-222, so as to minimize the effects of anaesthesia. Immunohistochemistry and imaging whole mounts Zebrafish were euthanized by icing, and then fixed in 4% paraformaldehyde (PFA) and 3% sucrose in 0.1 M phosphate-buffered saline (PBS), pH 7.4, for 25 min at room temperature. For anti-Gria2/3 (GluR2/3) immunohistochemistry, fish were fixed in 3% paraformaldehyde and 3% sucrose in PBS for 19 min at room temperature. Samples were washed three times for 5 min in PBS. Eyes were removed in PBS. Whole eyes were blocked in a solution containing 5% normal donkey serum and 0.5% Triton X-100 in PBS for 1–24 h and then incubated with primary antibodies. Primary antibodies included anti-GluR2/3 (rabbit, 1:300, Millipore), anti-ultraviolet opsin (rabbit, 1:500, kindly provided by David Hyde), anti-ultraviolet ospin (rabbit, 1:5,000, kindly provided by Jeremy Nathans), anti-blue opsin (rabbit, 1:5,000, kindly provided by Jeremy Nathans) and zpr-1 (mouse, 1:100, ZIRC) were diluted in blocking solution. After incubating in primary antibody for 1–3 days at 4 °C, samples were washed three times, 15 min each in 0.5% Triton X-100 in PBS and incubated for 3 h with secondary antibody, DyLight 649 Donkey anti-rabbit or anti-mouse (1:500, Jackson ImmunoReseach) diluted in blocking solution. After three, 15 min washes with 0.5% Triton X-100 in PBS, whole eyes were mounted in 0.5% agarose and coverslipped with Vectashield mounting medium (Vector). For H3 HC imaging, the eyes were oriented with the photoreceptor layer closest to the cover slip. For imaging of H3 HC dendritic tips with anti-GluR2/3 staining, eyes were hemisected by a scalpel blade (No.11, Feather) and mounted with the OPL perpendicular to the cover slip. Confocal image stacks were acquired on a FV1000 (Olympus) microscope using a 1.35 NA 60 × oil-immersion or 0.85 NA 20x oil-immersion objective lenses. Images were typically acquired with an XY resolution of 0.077 μm per pixel and 0.25 μm-thick Z slices for H3 HCs, and with an XY resolution of 0.462 μm per pixels and 1 μm-thick Z slices for whole eyes. Image analysis Stack images were median filtered in Matlab (Mathwork) and 3D-reconstructed in Amira (Mercury Computer Systems). To view the H3 HCs dendritic arbours in the ‘top view’, the 3D-reconstructed image was oriented with the OPL parallel to the viewing perspective. The ‘side view’ was generated by orienting the OPL perpendicular to the viewing perspective, and thinly sliced digitally using the oblique slice function in Amira. Dendritic tip invaginations into cones were determined by examining side views throughout the dendritic arbour of the HC. Connectivity maps were obtained by marking morphologically identified tip invaginations into cones on the maximum intensity projection of the H3 HC dendritic arbour. Dendritic field size and synapse distributions were measured from the connectivity maps using Fiji [53] . The locations of ultraviolet and blue cone terminal were marked on the connectivity maps and the total numbers of ultraviolet and blue cones within dendritic field were counted. The percentages of cones contacted within the dendritic field were obtained by dividing the number of ultraviolet or blue cones contacted by the total number of ultraviolet or blue cones within the dendritic field. Colabelling of transgenic fluorescent labels and immunofluorescence from anti-ultraviolet- or blue opsin staining was analysed using the masking function in Amira. Labelled cones were counted in Fiji using the maximum intensity projections of cells from Amira 3D reconstructions of whole eyes. Line scans of pixel intensity in Fig. 4 were obtained from side views of H3 HCs and cones using the MetaMorph (Universal Imaging) line scan function with 10-pt line thickness. Images in the figures were further processed in Photoshop (Adobe) by adjusting brightness, contrast and hues. Statistical analysis We used the Wilcoxon–Mann–Whitney rank sum test for comparisons of synapse numbers, dendritic field size, tip density, total tip number, percentage of cones contacted and ultraviolet/blue synapse ratios. ( Figs 1d , 3c , 5i–l , 6i–l , 8m–o , 9e–f , Supplementary Figs 1, 2b, 6 ) A one-way ANOVA was used to test for differences in the number of synapse across ages in Fig. 2b and for the dendritic field size in Fig. 3b . The Pearson correlation coefficient was calculated for the regression fit of the data points in Fig. 7d . Electron microscopy Briefly, zebrafish larvae were fixed in 4% glutaraldehyde in 0.1 M sodium cacodylate buffer, pH 7.4 for several hours, washed in buffer three times and placed in 1% osmium tetroxide in buffer. Tissue was dehydrated in a graded series of alcohol, embedded in resin, sectioned and imaged [19] . How to cite this article: Yoshimatsu, T. et al. Transmission from the dominant input shapes the stereotypic ratio of photoreceptor inputs onto horizontal cells. Nat. Commun. 5:3699 doi: 10.1038/ncomms4699 (2014).